Computational identification of a transiently open L1/S3 pocket for reactivation of mutant p53 The tumour suppressor p53 is the most frequently mutated gene in human cancer. Reactivation of mutant p53 by small molecules is an exciting potential cancer therapy. Although several compounds restore wild-type function to mutant p53, their binding sites and mechanisms of action are elusive. Here computational methods identify a transiently open binding pocket between loop L1 and sheet S3 of the p53 core domain. Mutation of residue Cys124, located at the centre of the pocket, abolishes p53 reactivation of mutant R175H by PRIMA-1, a known reactivation compound. Ensemble-based virtual screening against this newly revealed pocket selects stictic acid as a potential p53 reactivation compound. In human osteosarcoma cells, stictic acid exhibits dose-dependent reactivation of p21 expression for mutant R175H more strongly than does PRIMA-1. These results indicate the L1/S3 pocket as a target for pharmaceutical reactivation of p53 mutants. Tumour suppressor protein p53 is a transcription factor that has an important role in human cancers. It responds to various cell stress conditions, such as DNA damage, and controls pathways leading to apoptosis (programmed cell death), cellular senescence and cell cycle arrest, among others. Tumour initiation and maintenance depend upon inactivation of p53 pathways, which otherwise would deter uncontrolled cell growth. Consequently, p53 is the most frequently mutated gene in human cancers. Nearly half of all human tumours have mutant p53. Approximately three-quarters of those tumours that have mutant p53 are found to express full-length p53 protein with a single-residue missense mutation in the p53 DNA-binding core domain [1] , [2] . The resulting presence of full-length and single-point-mutated p53 protein in about one-third of all human tumours holds the promise of drugs that reactivate mutant p53 function, deter cancer cell proliferation, and shrink or kill the tumour [3] . Several p53-controlled pathways inhibit cell proliferation, and so are valid pharmaceutical targets. Studies on transgenic mice demonstrate that p53 reactivation enables tumour regression in vivo, even in advanced tumour cases [4] , [5] , [6] , [7] , [8] , [9] . Reactivation of p53 function has been demonstrated in various p53 cancer mutants by both second-site suppressor mutations [10] , [11] , [12] , [13] , [14] , [15] , [16] and a handful of small molecules [17] , [18] , [19] , [20] , [21] , [22] , [23] , [24] , [25] . The most well-studied and promising of these small molecules are PRIMA-1 and PRIMA-1 Met , currently in phase I/II clinical trials (APR-246-01, http://www.aprea.com/home/ ). PRIMA-1 is converted into several active products [26] , among them methylene quinuclidinone (MQ), that react covalently to alkylate p53 cysteine residues. This alkylation can reactivate p53 function [26] , although the precise reactivation mechanism remains elusive [27] . Here we describe computational analysis of p53 structural models that suggests a transiently open L1/S3 binding pocket around Cys124, Cys135 and Cys141 as a possible target for reactivation of p53 mutants by small molecules. The pocket was identified through genetic mutations, all-atom molecular dynamics (MD) simulations of the p53 core domain, computational solvent mapping of the resulting p53 structural ensemble and ensemble-based virtual screening. Mutation of Cys124 to alanine abolished known R175H reactivation effects of PRIMA-1 in human Saos-2 cancer cells. Ensemble-based virtual screening [28] , [29] was used to select 45 compounds with the most favourable predicting binding affinity to the L1/S3 pocket. Of these, stictic acid emerged as a p53 reactivation compound in cultured human osteosarcoma cells, with the ability to stabilize p53 in vitro . Computational identification of the L1/S3 binding pocket Initial docking of known p53 reactivation compounds (MQ, 3-methylene-2-norbornanone (NB), STIMA-1, MIRA-1, 2, 3 (refs 17 , 18 , 19 , 20 , 21 )) indicated preferential binding to a specific region in the mouse p53 core domain crystal structure (PDB ID 3EXJ [30] ), which has high sequence identity (~90%) to human p53. The corresponding region in the human p53 core domain is flanked by loop L1 and sheet S3 (hence, the L1/S3 pocket). The region had been labelled by genetic mutation studies [10] , [11] , [12] , [13] , [14] , [15] , [16] as highly enriched for p53 reactivation mutations ( Fig. 1 ; Phe113, Leu114, His115, Thr123, Leu137 and Asn235), indicating that subtle structural changes in this region can reactivate p53 cancer mutants. Four of those reactivation mutation sites (Phe113, Leu114, His115 and Thr123) plus Cys124 exhibit significant or moderate nuclear magnetic resonance (NMR) chemical shifts in response to binding of the p53-stabilizing peptide CDB3 (ref. 31 ). Cys124, Cys135 and Cys141 are near the centre of this putative p53 reactivation region, and covalent alkylation of a cysteine thiol group had been suggested for p53 reactivation by PRIMA-1 conversion products such as MQ and other p53 reactivation compounds [26] . 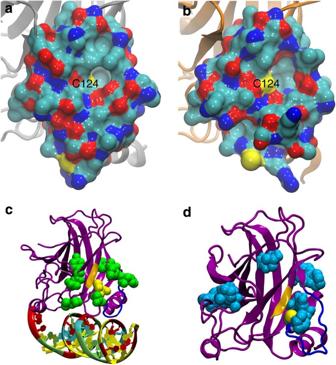Figure 1: Molecular visualizations of the p53 core domain. (a,b) All residues of the p53 core domain (1TSR-B33) within 10 Å of Cys124 are shown in a surface representation coloured by atom type: cyan, C; blue, N; red, O; yellow, S. (a) Cys124 is initially occluded in the wt crystal structure. (b) Structure extracted from MD simulations of mutant R273H reveals new breathing structural topography near Cys124 within the range of normal solution dynamics. (c,d) The p53 core domain is shown in magenta, loop L1 in blue, strand S3 in gold. (c) Cys124 (yellow) is surrounded by genetic mutation sites that can reactivate p53 function (green). (d) Druggable pockets (cyan) from FTMAP44for the R273H mutant. The open L1/S3 pocket surrounds Cys124 (yellow). In this cysteine triad, Cys124 was the most solvent-accessible, followed by Cys141 and then Cys135, in both the crystal structures and the MD simulations ( Table 1 ). Initial alkylation of Cys124 had been suggested to enable alkylation of Cys141 and then Cys135 (ref. 32 ). Figure 1: Molecular visualizations of the p53 core domain. ( a , b ) All residues of the p53 core domain (1TSR-B [33] ) within 10 Å of Cys124 are shown in a surface representation coloured by atom type: cyan, C; blue, N; red, O; yellow, S. ( a ) Cys124 is initially occluded in the wt crystal structure. ( b ) Structure extracted from MD simulations of mutant R273H reveals new breathing structural topography near Cys124 within the range of normal solution dynamics. ( c , d ) The p53 core domain is shown in magenta, loop L1 in blue, strand S3 in gold. ( c ) Cys124 (yellow) is surrounded by genetic mutation sites that can reactivate p53 function (green). ( d ) Druggable pockets (cyan) from FTMAP [44] for the R273H mutant. The open L1/S3 pocket surrounds Cys124 (yellow). Full size image Table 1 Summary of MD simulation trajectories and open pocket occurrences. Full size table In the crystal structures of the human p53 core DNA-binding domain (PDB IDs 1TSR [33] , 2OCJ [34] ), Cys124 is partially occluded and the putative L1/S3 reactivation pocket is not readily accessible to small molecules much larger than water. This occlusion in the crystal structure might seem to preclude alkylation of Cys124 in human p53. Blind docking of known p53 reactivation compounds onto the entire protein surface of the human p53 core domain crystal structure PDB ID 1TSR chain B (1TSR-B) [33] indicated that none of the compounds bound in close proximity to any cysteine, including those in the L1/S3 pocket ( Supplementary Fig. S1 ). However, the L1 loop can undergo a conformational switch to regulate DNA binding by an induced fit mechanism [35] , [36] . NMR studies demonstrate that Cys124 is exposed to solvent ~5% of the time [37] . Mass spectrometry results indicate that Cys124 and Cys141 react preferentially with alkylating agents [32] and with glutathione [38] . Alkylating agents cause NMR chemical shifts of several residues within the L1/S3 region [32] , including Leu114, His115 and Thr123, already implicated above by genetic mutations and CDB3-induced NMR chemical shifts. Wild-type p53 is marginally stable at physiological temperature. The DNA binding domain unfolds with a half-life of around 9 min 3 and has a low melting temperature ( T m ) of about 36–46 °C depending on experimental conditions [39] , [40] , [41] . All-atom explicit solvent MD simulations for 30 ns of wild-type p53 and three frequent cancer mutants, R175H, G245S and R273H, revealed a high degree of flexibility for the core domain [42] and particularly the L1/S3 region surrounding Cys124 ( Supplementary Movie 1 ). Clustering the MD ensembles with respect to the L1/S3 pocket conformation further demonstrated the flexibility of the region ( Table 1 ). In the MD ensembles of different p53 variants, average solvent-accessible surface area (SASA) values of the Cys124 side chain were calculated to be in the range of 6–11 Å 2 ( Table 1 ). In sharp contrast, in the p53 core domain crystal structure 1TSR-B the Cys124 side chain SASA was calculated to be only 0.43 Å 2 . Docking into the L1/S3 pocket A transiently open L1/S3 pocket formed around Cys124 due to positional and conformational changes of Ser116, Thr123, Cys124, Thr140 and especially Leu114 ( Fig. 1 ). Three of these residues, Leu114, Thr123 and Cys124, already were implicated above. We determined five distance/dihedral angle criteria ( Supplementary Methods ) that indicated formation of an open L1/S3 pocket in about 5–8% of each simulation ( Table 1 ). Fpocket [43] , a program to measure the volume of a defined binding pocket ( Fig. 1 ), also identified an open L1/S3 pocket around Cys124 across several p53 variants in 5–30% of the 3,000 frames of each MD trajectory ( Table 1 ). For evaluating Fpocket results, the L1/S3 pocket was considered open if its volume was >150 Å 3 , a lower bound chosen based on cancer mutant R273H, which exhibited the lowest average L1/S3 pocket volumes. FTMap [44] , a program to identify ligand-binding hot spots in proteins using organic solvent probes, predicted the L1/S3 pocket to be among the most highly occupied by the solvent probes when used to assess druggability of MD-generated conformations ( Fig. 1 ). For wt p53 and mutant R273H MD trajectories, FTMap predicted a druggable L1/S3 pocket to occur, respectively, in 11 and 7 of the 15 most-populated cluster centroids. In contrast, neither Cys124 nor any other cysteine in the original PDB crystal structure 1TSR-B [33] was identified as a druggable site by FTMap. Several previously identified alkylating p53 reactivation compounds, MQ [26] , NB [21] , STIMA-1(ref. 22 ) and MIRA-1, 2, 3 (ref. 19 ), subsequently were docked into the most-populated MD trajectory cluster representative that had an open L1/S3 binding pocket as defined ( Table 1 , Supplementary Methods ). All of these known active compounds presented low-energy predicted docking poses with the reactive methylene oriented in close proximity to the Cys124 sulphydryl group for p53 cancer mutant R175H ( Fig. 2 ). Supplementary Fig. S2 depicts the corresponding ligand interaction diagrams, and Supplementary Table S1 provides the corresponding docking statistics. Reliability of the molecular docking strategy was supported by a positive control, PhiKan083 (ref. 23 ), which docked within 1.0 Å root-mean-square-deviation (RMSD) of the reference crystal structure ( Supplementary Fig. S1 ). The transiently open L1/S3 pocket was shared across wild-type and the three p53 cancer mutants studied ( Supplementary Fig. S3 ). Thus, several lines of evidence suggested a transiently open and druggable binding pocket in the L1/S3 region of the human p53 protein. 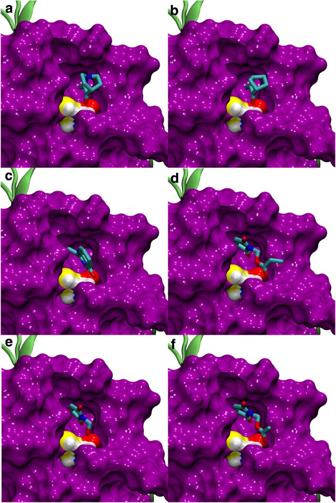Figure 2: Known p53 reactivation compounds docked into the open L1/S3 pocket of R175H. (a) MQ (from PRIMA-1)26, (b) NB21, (c) STIMA-1 (ref.22,d) MIRA-1 (ref.19,e) MIRA-2 (ref.19,f) MIRA-3 (ref.19). Known p53 reaction compounds could dock favourably into the most-populated R175H MD trajectory cluster centroid that had an open L1/S3 pocket. All of the nine docking poses generated by Autodock Vina for each compound above scored within the published standard error of Autodock Vina docking scores60(Supplementary Table S1). In each case, the binding pose depicted above had the smallest distance between the reactive methylene of the small molecule and the Cys124 sulphydryl group. The protein surface representation is purple, except Cys124 atoms are coloured by atom type as in Fig. 1a,b. Figure 2: Known p53 reactivation compounds docked into the open L1/S3 pocket of R175H. ( a ) MQ (from PRIMA-1) [26] , ( b ) NB [21] , ( c ) STIMA-1 (ref. 22 , d ) MIRA-1 (ref. 19 , e ) MIRA-2 (ref. 19 , f ) MIRA-3 (ref. 19 ). Known p53 reaction compounds could dock favourably into the most-populated R175H MD trajectory cluster centroid that had an open L1/S3 pocket. All of the nine docking poses generated by Autodock Vina for each compound above scored within the published standard error of Autodock Vina docking scores [60] ( Supplementary Table S1 ). In each case, the binding pose depicted above had the smallest distance between the reactive methylene of the small molecule and the Cys124 sulphydryl group. The protein surface representation is purple, except Cys124 atoms are coloured by atom type as in Fig. 1a,b. Full size image Biological validation of the L1/S3 binding pocket hypothesis We examined the role of Cys124 in the L1/S3 binding pocket by site-directed mutagenesis of Cys124 to alanine (C124A). If Cys124 were a critical residue for p53 reactivation, then removal of its thiol group by this otherwise innocuous mutation would abolish the PRIMA-1 reactivation effect. For example, Cys124 might be a key attachment residue for PRIMA-1 conversion products such as MQ [26] , it might initiate a Cys124-Cys141-Cys135 alkylation cascade [32] , or it might form a disulphide bond that stabilized p53 in an active conformation induced by compound binding. The literature suggests that a reducing environment leads to correct p53 folding and disulphide bond formation may lead to aggregation [27] . There is no a priori reason to rule out any of these hypotheses. p53 null human osteosarcoma Saos-2 cells were engineered to have doxycycline-inducible expression of either wild-type p53 or various p53 mutants. Single clones with similar expression levels of the different p53 variants were selected for direct comparison of small-molecule effects ( Supplementary Fig. S4 ). As expected, expression of wild-type p53 in Saos-2 cells halted cell proliferation, whereas expression of mutant R175H had no effect on cell proliferation ( Fig. 3 ). Mutation of Cys124 to alanine had little effect on otherwise wild-type p53 (C124A) nor did it restore activity of R175H (R175H_C124A), indicating that the C124A mutation is largely neutral for general p53 function. Consistent with previous results [26] , addition of PRIMA-1 to cells expressing inactive mutant R175H led to p53 reactivation and subsequent inhibition of cell cycle progression. Importantly, PRIMA-1 reactivation of p53 function was blocked in the double mutant R175H_C124A ( Fig. 3 ), demonstrating the importance of Cys124 in pharmacological reactivation of mutant R175H by PRIMA-1. These experimental results supported the computational identification of the L1/S3 binding pocket surrounding Cys124 as significant for p53 reactivation. 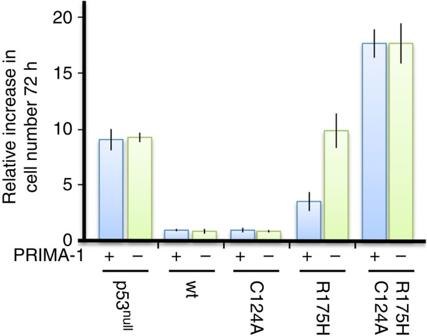Figure 3: PRIMA-1 acts through cysteine 124 in p53. p53nullSaos-2 cells expressing wild-type p53, or the indicated p53 mutants, were treated with 50 μM preheated PRIMA-1 (blue bar) or the medium without PRIMA-1 (DMSO, green bar) for 72 h. The increase in cell number during 72 h of growth is shown. The s.d. represent four independent samples. Figure 3: PRIMA-1 acts through cysteine 124 in p53. p53 null Saos-2 cells expressing wild-type p53, or the indicated p53 mutants, were treated with 50 μM preheated PRIMA-1 (blue bar) or the medium without PRIMA-1 (DMSO, green bar) for 72 h. The increase in cell number during 72 h of growth is shown. The s.d. represent four independent samples. Full size image L1/S3 pocket identifies a novel p53 reactivation compound An ensemble-based virtual screening approach, known as the relaxed complex scheme [28] , [29] , was performed against the mutant R273H. Initially, 1,324 compounds from the NCI/DTP Open Chemical Repository Diversity Set II were virtually screened (The NCI/DTP Open Chemical Repository, http://dtp.cancer.gov ). They were docked into each of the most-populated 15 cluster centroids—altogether representing 92.5% of the entire trajectory—obtained by clustering the MD trajectory of the R273H cancer mutant according to the L1/S3 pocket conformation. Compounds with predicted binding affinities of −6.5 kcal mol −1 or better to any of the 15 centroids were chosen with a limit of 50 compounds from each centroid. The resulting 84 compounds (corresponding to ~6% of the entire NCIDS2 database) were ranked according to their population-weighted average binding affinities. The absorption, distribution, metabolism, and excretion (ADME) properties of the compounds, as predicted by Schrodinger (QikProp, version 3.3, Schrödinger, LLC, New York, NY, 2010), were used for further filtering. Lipinski’s Rule of Five and Jorgensen’s Rule of Three were followed strictly, resulting in 24 compounds. Similarly, compounds from the NCI Mechanistic Set, NCI Natural Products Set, NCI COMBO Set, and NCI Oncology-Approved Set (consisting of 974 compounds in total) were virtually screened and filtered for ADME properties. A more stringent ADME filter (octanol/water partition coefficient <3) was enforced to improve compound solubility. A similar predicted binding affinity cutoff of −6.5 kcal mol −1 was used, resulting in 24 additional compounds. Three selected compounds were discarded because they were unavailable (NSC-653010, NSC-92339 and NSC-653016). In total, 45 compounds were selected for biological assay ( Supplementary Tables S2 and S3 ). One of these compounds, stictic acid (NSC-87511), proved to be a p53 reactivation compound. 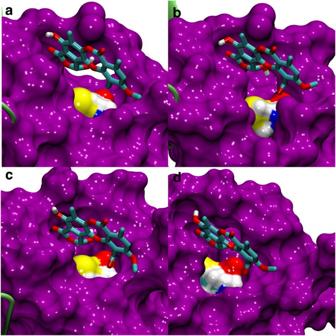Figure 4: Stictic acid docked into open L1/S3 pocket of p53 variants. Stictic acid could dock favourably into the open L1/S3 pocket of MD-generated snapshots for all four p53 variants studied: (a) wt p53; (b) R175H; (c) R273H; (d) G245S. Only polar hydrogens of stictic acid are depicted here. Colours are as in Fig. 2. Figure 4 illustrates the best-scoring stictic acid pose when docked into the L1/S3 pockets of wt p53 and mutants R175H, R273H and G245S. Supplementary Figure S5 shows how stictic acid ranked on a histogram of best docking scores of the screened compounds using mutant R273H, and Supplementary Fig. S6 compares docking scores between mutants R273H and R175H (correlation coefficient=0.80). The predicted binding affinities, z -scores, mean and standard deviation for the nine docked poses of stictic acid with mutant R175H are presented in Supplementary Table S1 . To gauge the stability of stictic acid in the L1/S3 active site, a MD simulation was performed starting from the best-scoring docking pose of stictic acid in mutant R175H. The initial docking score was −6.97 and the final docking score was −7.11. Supplementary Figures S7 and S8 show that the p53 core domain was stable and stictic acid persisted in the L1/S3 pocket throughout the entire 60 ns MD simulation. Supplementary Figure S9 compares the poses and detailed molecular interactions of stictic acid docked to mutant R175H in the docked pose of Fig. 4b and again after 60 ns of MD simulation. Figure 4: Stictic acid docked into open L1/S3 pocket of p53 variants. Stictic acid could dock favourably into the open L1/S3 pocket of MD-generated snapshots for all four p53 variants studied: ( a ) wt p53; ( b ) R175H; ( c ) R273H; ( d ) G245S. Only polar hydrogens of stictic acid are depicted here. Colours are as in Fig. 2. Full size image Experimental support for stictic acid and p53 reactivation Stictic acid partially restored p53 activity in human Saos-2 cells expressing cancer mutant R175H ( Fig. 5 ), as demonstrated by induction of the cell cycle inhibitor p21. p21 is a canonical gene target of active p53 and a sensitive and selective output for p53 activity. Induction of p21 by stictic acid was dose-responsive, as shown in Fig. 5 . It was also dependent upon p53, because it had only a minor effect on p21 expression in cells lacking p53 ( Fig. 5 , Supplementary Fig. S4 ). 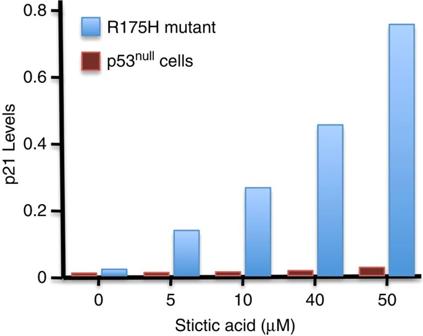Figure 5: Dose-dependent p21 activation in response to stictic acid. Saos-2 cells (p53null) and Saos-2 cells stably expressing the p53 cancer mutant R175H were treated with doxycycline for 8 h to induce expression of mutant R175H. Cells were then grown for 48 h in the presence of stictic acid at the concentrations indicated. p21 expression was quantified using a Fuji LAS-4000 imaging system and plotted normalized to the expression of tubulin in each sample. Figure 5: Dose-dependent p21 activation in response to stictic acid. Saos-2 cells (p53 null ) and Saos-2 cells stably expressing the p53 cancer mutant R175H were treated with doxycycline for 8 h to induce expression of mutant R175H. Cells were then grown for 48 h in the presence of stictic acid at the concentrations indicated. p21 expression was quantified using a Fuji LAS-4000 imaging system and plotted normalized to the expression of tubulin in each sample. Full size image p53 primarily functions as a transcriptional activator. To test more directly the effect of stictic acid on restoring transcriptional activator function of p53 mutants we generated stable cell lines harbouring reporter constructs driven by two different p53-dependent promoter elements. These elements were derived from the promoters of the cell cycle inhibitor p21 and the proapoptotic gene PUMA and have previously been utilized to monitor p53 transactivation activity [45] . We compared the effect of stictic acid to that of PRIMA-1 and the recently identified allele-specific p53 reactivation compound NSC-319725 ( [25] ; Fig. 6 ). All compounds modestly but significantly restored the ability of the p53 mutants R175H and G245S to express the proapoptotic reporter PUMA, except NSC-319725, which acted in an mutant-specific manner as expected [25] ( Fig. 6a ). Activation of p21 reporter transcription was more pronounced and confirmed that stictic acid is a p53 mutant reactivation compound comparable to previously identified compounds. 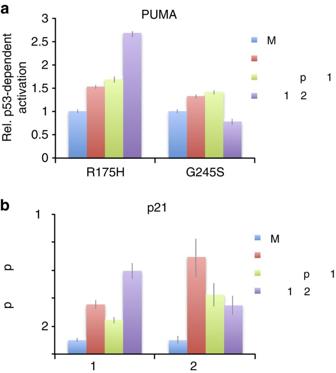Figure 6: p53-dependent activation of PUMA and p21 transcription reporter by reactivation compounds. Preheated26PRIMA-1 (25 μM), NSC-319425 (25 μM) and stictic acid (10 μM) were added to stable Soas-2 (p53null) cell lines harbouring (a) PUMA- or (b) p21-dependent luciferase reporter and expressing the p53 mutants R175H or G245S as indicated. Activation of PUMA and p21 transcriptional reporter was measured by luciferase activity assays. Reporter cell lines without p53 expression were processed in parallel and used for normalization to visualize p53-dependent effects. Data are represented as mean±s.d. (n=4). Figure 6: p53-dependent activation of PUMA and p21 transcription reporter by reactivation compounds. Preheated [26] PRIMA-1 (25 μM), NSC-319425 (25 μM) and stictic acid (10 μM) were added to stable Soas-2 (p53 null ) cell lines harbouring ( a ) PUMA- or ( b ) p21-dependent luciferase reporter and expressing the p53 mutants R175H or G245S as indicated. Activation of PUMA and p21 transcriptional reporter was measured by luciferase activity assays. Reporter cell lines without p53 expression were processed in parallel and used for normalization to visualize p53-dependent effects. Data are represented as mean±s.d. ( n =4). Full size image Differential scanning fluorimetry (DSF) provides the ability to detect molecular interactions between a small molecule and a protein based on changes in the melting temperature ( T m ) of the protein [46] . These T m changes are taken to reflect changes in protein stability upon binding of the small molecule. Variants of the p53 core domain (wild type, G245S and R175H) were tested in DSF assays with a range of concentrations of PRIMA-1, MQ and stictic acid ( Fig. 7 ). The T m values in the absence of compounds for wild type, G245S and R175H, at 4 μM, were 36.54±0.11, 33.51±0.09 and 27.89±0.11 °C, respectively. PRIMA-1 and MQ stabilized each of the p53 variants by ~≤1° for concentrations ranging from 10 to 80 μM, 2.5 × to 20 × stoichiometric ratio of compound to protein ( Fig. 7 ). The greatest thermal stabilization was observed with stictic acid, up to 4.60±0.39 °C at 80 μM in mutant R175H. All three of these compounds demonstrated a relative dose dependence in their ability to stabilize p53. None of these compounds had stabilizing effects on three control proteins tested, annexin A2, S100A4 and S100A10, suggesting that their interactions are specific to p53. 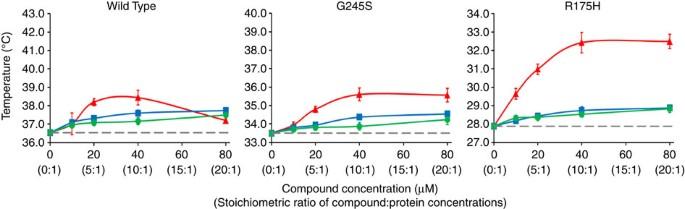Figure 7: Thermal stabilization of p53 mutants by reactivation compounds. Selected concentrations of PRIMA-1 (blue, square), MQ (green, circle) and stictic acid (red, triangle) were added to 4 μM of wild type, G245S and R175H core domain protein. Thermal stabilization was measured using DSF. Data points are plotted as the mean of sextuplet measurements, with corresponding 95% confidence intervals. Confidence interval bars not visible are smaller than the symbol used to plot the data point. PRIMA-1 and MQ stabilized each p53 variant about 1 °C or less over this range of concentrations. Stictic acid resulted in the greatest stabilization for both p53 mutants studied. Figure 7: Thermal stabilization of p53 mutants by reactivation compounds. Selected concentrations of PRIMA-1 (blue, square), MQ (green, circle) and stictic acid (red, triangle) were added to 4 μM of wild type, G245S and R175H core domain protein. Thermal stabilization was measured using DSF. Data points are plotted as the mean of sextuplet measurements, with corresponding 95% confidence intervals. Confidence interval bars not visible are smaller than the symbol used to plot the data point. PRIMA-1 and MQ stabilized each p53 variant about 1 °C or less over this range of concentrations. Stictic acid resulted in the greatest stabilization for both p53 mutants studied. Full size image Despite continuous progress in cancer research and care, millions of people die annually from this disease. Therapeutic reactivation of p53 could prevent or delay many of these deaths. The p53 Y220C reactivation pocket already has been used for rational drug design and discovery in that specific mutation [23] , [24] . Here we report computer-guided identification of a transiently open L1/S3 reactivation pocket in p53 that may present a more broadly applicable druggable region for such cancer therapies. The coordinates of the human p53 core domain structures with the open binding pocket conformations shown in Fig. 4 appear as Supplementary Data S1 , and also have been deposited in the Protein Model DataBase (PMDB) [47] ( http://mi.caspur.it/PMDB/ ; PMDB ID (a) PM0078199 for wt p53; (b) PM0078200 for R175H; (c) PM0078201 for G245S; and (d) PM0078202 for R273H) and in SourceForge ( http://sourceforge.net/projects/p53cancerrescue/ , in folder ‘Coordinates of p53 core domain’). We anticipate that the L1/S3 reactivation region reported here will be useful to other researchers carrying out structure-based drug discovery and development of p53 reactivation drug leads. A notable advantage of the L1/S3 pocket is that it occurs across several p53 variants, as seen in Fig. 4 and Supplementary Figs S3 and S6 , giving hope that p53 reactivation compounds can be developed to target several p53 cancer mutants simultaneously. In contrast, for example, known compounds that target the p53 Y220C reactivation pocket [23] , [24] may be specific to the Y220C mutant, because specific structural details of the Y to C mutation were used in their design or discovery. None of the R175H, G245S or R273H mutations lie in the L1/S3 pocket or have direct effects on its conformation. Its generalizability is illustrated here by the result that virtual screening against one mutant, R273H, produced a compound that resulted in biological validation against a different mutant, R175H, and induced DSF temperature shifts in all p53 variants studied. Protein conformational flexibility is well-recognized as an important factor in ligand binding. A few computational drug discovery approaches attempt to accommodate protein-induced fit on ligand binding by allowing side chains to move to improve the fit of the ligand into the binding pocket. Very few such approaches allow the protein backbone to move to accommodate the ligand. Nevertheless, the results above provide a cautionary tale: a ligand-binding pocket of medical importance may be hidden and difficult to recognize in structural databases, yet other virtual structures extracted from its conformational ensemble may support successful structure-based drug discovery. With appropriate protein conformations in hand for computational analysis, we screened only 45 compounds through biological assays to find a novel p53 reactivation compound, stictic acid. Our relaxed complex scheme [28] , [29] clusters are based on conformations of all residues surrounding the L1/S3 pocket, not on specific conformations of particular residues. No cluster centroid produced a suitable docking pose for stictic acid docked to G245S ( Fig. 4d ), due to the position and rotamer state of the crucial Leu114 residue. A suitable Leu114 conformation occurred in only three or four frames of the entire 3,000-frame 30-ns trajectory (Methods, RMSD-based clustering). The sampling in MD is limited, so the fact that any suitable pocket-opening events were seen at all is indication that such pockets exist at thermal equilibrium for this mutant. Indeed, three occurrences in 30 ns is equivalent to 10 8 occurrences per second, whereas three occurrences in 3,000 frames is equivalent to a probability of 10 −3 , and so the event cannot be considered rare. Instead, we see here a limitation of our current computational methods for modelling complex molecular processes. As seen in Supplementary Figs S7 and S9 , stictic acid remained docked after 60 ns of stable MD simulation. The rotamer state of Leu114 was critical to opening up a binding site large enough to accommodate large molecules such as stictic acid. In the initial docked pose of stictic acid ( Supplementary Fig. S9a ), there is only one direct H-bond interaction between stictic acid and the Cys124 backbone amino group, in addition to various hydrophobic interactions including Pro142 and Leu114 ( Supplementary Fig. S9c ). The hydrophobic interactions with Pro142 and Leu114 were conserved throughout the simulation. The final pose ( Supplementary Fig. S9b ) provides an elegant illustration of induced fit upon binding. Stictic acid moved deeper into the pocket, achieved a very nice shape complementarity, substantially expanded the initial network of favourable direct and water-mediated interactions, and shifted the ligand and receptor exposure patterns ( Supplementary Fig. S9d ). PRIMA-1 has conversion products that are more active than it is itself [26] , and this may be the case for stictic acid as well. The existence of a highly active and bioavailable stictic acid decomposition product was suggested by initial experiments carried out with a stictic acid solution that had a long storage time. Such hypothetical conversion products were not present in the freshly ordered newly dissolved pure compound, from which the results presented here were derived. It is unclear whether or not stictic acid requires covalent linkage to p53 for reactivation according to the general cysteine alkylation mechanism proposed by Lambert et al. [26] for several other p53 reactivation compounds. Stictic acid may, in principle, bind covalently to nucleophilic protein side chains by acylating or alkylating nucleophilic residues such as cysteine. Likely reaction sites and modes of reactivity ( Supplementary Fig. S10 ) include the direct addition of a nucleophile (a cysteine thiol group of the protein, as represented in the figure) to either the seven-membered ring lactone carbonyl group (A) or to the carbonyl group of the five-membered ring lactone (B), resulting in acylation of the thiol and covalent attachment to the protein as the respective thioester. Alkylation is another possible mechanism, occurring via a more circuitous mechanism (C) in which dehydration generates a reactive quinone methide-type species that can alkylate nucleophiles, as illustrated schematically for a p53 cysteine side chain thiol group. An alternative dehydration pathway (loss of a proton on the para-methyl group, not shown) could produce a different methide that would result in alkylation at the corresponding benzylic position. There is no a priori reason to rule out any of these pathways. In DSF experiments, preheated PRIMA-1 (to induce formation of conversion products [26] ) induced thermal shifts ( T m increases) that were slightly higher than that for MQ. Though slight, the differences were statistically significant at higher concentrations, which is consistent with the previous evidence that MQ is not the most active conversion product of PRIMA-1 (ref. 26 ). These two known reactivation compounds showed significantly lower stabilizing effects on the p53 mutants tested than did stictic acid. Stictic acid is a much larger molecule than MQ. It has the potential to make more interactions within the binding pocket (compare Figs 2 with 4 ,), perhaps giving it a greater capacity than PRIMA-1 or MQ for stabilizing p53 cancer mutants. We cannot rule out other effects, for example, the possibility that the low thermal shifts for PRIMA-1 may be due to its incomplete conversion into more active products, or that the low thermal shifts for MQ may be due to its highly reactive nature leading to rapid decomposition on contact with water. Stictic acid displayed promising results in reactivating severely destabilized mutant R175H in human cancer cells. Reactivation was evident from dose-dependent and p53-dependent induction of p21 expression. Cell death was not activated by stictic acid, which may be due to insufficient reactivation of cancer mutant R175H or may indicate pathway-selective restoration of p53 activity. Such probes with pathway discriminatory activity will become valuable tools for the study of p53 biology. PUMA reporter assays demonstrated comparable p53 reactivation by stictic acid and PRIMA-1 ( Fig. 6 ), yet PRIMA-1 is a potent inducer of apoptosis in cells with mutant p53. It is possible that additional, p53-independent cytotoxic functions of PRIMA-1 or one of its degradation products [26] act synergistically with p53 reactivation to induce apoptosis. Such additive effects may not be induced by stictic acid. Mutant R175H showed a greater degree of thermal stabilization in DSF by stictic acid than did wild type or G245S. Perhaps, this is because R175H is initially highly destabilized (a Zn region mutant, 30% folded at 37 °C [40] ) while wild type and G245S (a DNA region mutant, 95% folded at 37 °C [40] ) are not. These results indicate that stabilization effects and reactivation outcome depend on the p53 mutation, and that thermal stabilization of the p53 core domain may reactivate some p53-controlled pathways and not others in a way that depends on the ligand. DSF in vitro experiments indicated direct binding of stictic acid to all p53 variants tested. Induction of p21 expression by stictic acid showed dependence on p53-mediated pathways, because no such induction was observed in the Saos-2 parent cell lines lacking p53. Taken together, these in vitro and in cellulo results indicate that stictic acid acts directly on p53. Recently, two compounds from the thiosemicarbazone family (for example, NSC-319725) were identified as allele-selective reactivation compounds for p53 cancer mutant R175H [25] . Whether these compounds directly bind to p53 and target the L1/S3 reactivation pocket identified in this study is currently unclear, but will be interesting questions to address in future experiments. Our results demonstrate the value of integrated strategies combining genetics and computation for identification of druggable protein regions, and highlight the feasibility of using MD simulations to expose druggable protein regions that otherwise may not be evident. MD simulations Wild-type p53 MD simulations were performed using crystal structure 1TSR-B [33] for the initial coordinates. Models for mutants R273H, R175H, G245S and C124A were prepared by virtual mutation of wild-type p53 using the AMBER10 suite [48] . The crystallographic water molecules were retained and each system was solvated in a TIP3P water box [49] . Zinc-coordinating residues were modelled using the cationic dummy atom model [50] . Protonation states of titratable residues were determined using the Whatif Web Interface [51] . Histidine, asparagine and glutamine side chain orientations were corrected as needed using the Molprobity web server [52] . Each system was neutralized by adding chloride ions as needed. The structure files of each system consisted of about 27,260 atoms, which were prepared using the AmberFF99SB force field [53] . Each of the p53 variant systems was first relaxed using 36,000 steps of minimization followed by four consecutive restrained 250 ps MD simulations. Thereafter, 30 ns unrestrained MD simulation was performed at 310 K and 1 atm for each system using the NAMD2.7 suite [54] . Details of the minimization and MD simulation protocol can be found in Demir et al. [42] To gauge the stability of the stictic acid in the binding pocket, a 60 ns MD simulation was performed. The best-scoring docked pose of the molecule in the R175H L1/S3 open-pocket conformation was used as the starting geometry ( Fig. 4b , Supplementary Table S1 ). Stictic acid parameters were generated with the Antechamber module of Amber10 using the Generalized Amber Force Field [55] , [56] with RESP HF 6-31G* charges. For each p53 variant studied, the solvent-accessible surface area of the Cys124 side chain over the MD trajectory was calculated using a customized visual molecular dynamics [57] (VMD) script. The coordinates of the human p53 core domain structures with the open-binding pocket conformations shown in Fig. 4 appear as Supplementary Data S1 , and also have been deposited in the PMDB 47 ( http://mi.caspur.it/PMDB/ ; PMDB ID (a) PM0078199 for wt p53; (b) PM0078200 for R175H; (c) PM0078201 for G245S; and (d) PM0078202 for R273H) and in SourceForge ( http://sourceforge.net/projects/p53cancerrescue/ , in folder ‘Coordinates of p53 core domain’). RMSD-based clustering Protein snapshots extracted from the simulations were clustered with respect to all heavy atoms of the L1/S3 site. For each variant, atomic coordinates were extracted at 10 ps intervals over their 30 ns MD trajectory, resulting in 3,000 simulated structures per trajectory. These 3,000 structures were superimposed with respect to all C α atoms to remove overall translation and rotation. They were then clustered using the gromos algorithm [58] in the GROMACS 4.0.5 program [59] at an RMSD cutoff value of 1.65 Å, based on atomic coordinates of all atoms of those residues that had at least one atom within 10 Å of Cys124 in the minimized and equilibrated form of each p53 variant. In each cluster, the structure with the smallest average RMSD to all the other structures in the cluster was designated as the ‘centroid’ or ‘representative’ structure of the cluster. Cluster centroids exhibiting open L1/S3 pockets were identified for each p53 variant using the geometric criteria ( Supplementary Methods ). These open centroids were used for docking stictic acid and the known p53 reactivating small molecules. In the case of G245S, the known small molecules were successfully docked into the cluster centroid with an identified open L1/S3 pocket. However, it was not possible to identify a cluster centroid for G245S that produced a binding pose for stictic acid (a relatively much larger molecule) in which a possible alkylation reaction with the Cys124 side chain seemed reasonable. A closer look at the G245S MD trajectory revealed that the position and rotamer state of Leu114 was critical for L1/S3 pocket opening. Leu114, already implicated above, exhibited a favourable conformation in only three or four frames of the entire 3,000-frame trajectory. Thus, a snapshot with an open L1/S3 pocket was extracted manually from the G245S MD trajectory and subsequently used to dock stictic acid. In silico docking Initial docking studies were performed using AutoDock 4.2.2 (SMILES strings for all small molecules considered explicitly in this paper are given in Supplementary Table S4 ). All subsequent docking studies used AutoDock Vina [60] with an exhaustiveness value of 100 and a 20 × 20 × 20 Å search space centred on the sulphur atom of Cys124. Nine different docking poses were calculated for each considered combination of a compound and a p53 variant. For initial compound scoring, population-weighted average binding affinities of the most-populated 15 cluster centroids from the R273H MD trajectory were calculated using the best binding affinity found by Autodock Vina for each compound. The 48 compounds selected were re-scored using the population-weighted average binding affinities of the most-populated 30 cluster centroids. Ligand interaction diagrams were prepared using the Molecular Operating Environment program (Chemical Computing Group Inc., Montreal, Canada). Computational fragment mapping using FTMap The FTMap program [44] utilizes 16 probe molecules to identify and rank the most energetically favourable binding pockets on a protein surface. For this purpose, FTMap first performs rigid body docking of probe molecules with a fast Fourier transform method, then minimizes and rescores the docked poses. Next, it clusters them for each probe using a simple greedy algorithm, and finally locates the consensus sites of binding pockets identified by all probes. Cell lines Soas-2 cells were obtained from the American Type Culture Collection (Manassas, VA, USA). They were maintained at 37 °C in DMEM high glucose supplemented with 10% FBS, penicillin G sodium (100 units ml −1 ) and streptomycin (100 μg ml −1 ). Stable Soas-2 cell lines harbouring doxycycline-inducible p53 wild type or mutants were established by a lentivirus-based strategy. Human p53 genes were cloned as Sac I/ Pst I fragments into pEN_TmiRc3, replacing GFP and ccdB genes in the plasmid. Recombination of p53-pEN_TmiRc3 and the lentivirus vector pSlik was performed using the LR Clonase Enzyme Mix (Invitrogen, Carlsbad, CA) according to manufacturer’s instructions. Lentiviruses were generated by co-transfecting 5 μg of lentiviral vector pSlik and 5 μg of each packaging vector (coding for Gag, Pol, Tat, Rev and VSVG) in 90% confluent 293T cells in 10-cm plates using Lipofectamine 2000 (Invitrogen, Carlsbad, CA). Supernatants were collected 48 h after transfection and used directly to infect Soas-2 cells. Forty-eight hours after this infection, the Soas-2 cultures were switched to hygromycin B-containing media. To isolate single p53-expressing clones, cells were induced with doxycycline and tested by immuno blotting. Doxycycline was used at a concentration of 1 μg ml −1 , hygromycin B at 50 μg ml −1 . For generation of stable cell lines to measure p53-dependent activation of p21 or PUMA reporters, p21 (5′-GAAGAAGACTGGGCATGTCT-3′) or PUMA (5′-CTGCAAGTCCTGACTTGTCC-3′) response elements [45] followed by a minimal promoter (5′-TAGAGGGTATATAATGGAAGCTCGACTTCCAG-3′) were inserted into Kpn I/ Xho I cut plasmid pGL4.10 (Promega). These elements control the expression of a synthetic firefly luc2 ( Photinus pyralis ) gene. A SV40-driven puromycin resistance cassette was inserted into the Pst 1 site of pGl4.10 to enable generation of stable cell lines. The PUMA and p21 reporter vectors were transfected into Soas-2 cells and single colonies resistant to 50 μg ml −1 puromycin were selected. Cell viability assay Cells were placed in 96-well plates at a density of 10,000 cells per well and incubated overnight. The next day, doxycycline (final concentration 1 μg ml −1 ) was added to induce the expression of p53 for 8 h before PRIMA-1 (50 μM final concentration) or solvent was added to the cultures. PRIMA-1 was preheated to 100 °C for 10 min to promote formation of active decomposition products and then cooled before it was used in these experiments [26] . Cell viability assays were performed using CellTiter-Glo Luminescent Cell Viability Assay (Promega, Wisconsin, MD) according to the manufacturer’s instructions. Data represent the average of four independent samples. Western blot analysis Approximately 500,000 cells were treated with doxycycline at a final concentration of 1 μg ml −1 for 8 h to induce expression of p53, then treated with stictic acid or vehicle (dimethylsulphoxide, DMSO) at various concentrations for 48 h. For western blot analysis, cells were lysed in 8 M Urea buffer and equal amounts of total cell lysates were resolved by SDS–PAGE (12.5% gel). Then proteins were transferred onto Immobilon PVDF membrane (Millipore) and probed with an anti-p21 antibody (Santa Cruz Cat#: sc-397). p21 expression was quantified using a Fuji LAS-4000 imaging system and analysed with the Multi Gauge v3 software. PUMA and p21 reporter assay Soas-2-PUMA-luc2 or Soas-2-p21-luc2 cell lines were transfected with 500 ng of cytomegalovirus-renilla plasmid and 125 ng of plamid carrying either empty vector, p53 wt or mutants R175H and G245S [12] using Lipofectamine 2000. The different compounds were added 21 h after transfection. Activation of the PUMA and p21 reporters was analysed by a luciferase assay (Dual luciferase assay system, Promega) 8 h after the addition of compounds. Purification of wild-type and mutant p53 core domains The wild-type p53 core domain (residues 94-312) had been previously introduced into the bacterial expression vector pSE420. Mutants G245S and R175H were generated by using a site-directed mutagenesis kit in this same vector (Invitrogen, Grand Island, NY). These vectors were transformed into Escherichia coli Rosetta 2 (DE3) strain, then expressed as described [34] . Proteins were purified in a series of chromatographic steps: Q-Sepharose anion exchange column, SP-Sepharose cation exchange column, affinity chromatography using a HiTrap heparin Sepharose column and gel filtration on a Superdex 200 column (GE Healthcare, Piscataway, NJ), followed by dialysis against 50 mM HEPES pH 7.5, 150 mM NaCl and 0.1 mM dithiothreitol. Pure protein was concentrated by Macrosep Advance Centrifuge Devices (PALL, Port Washington, NY) to 0.22 mM and stored at −20 °C for further use. Protein concentration was determined by a Shimadzu (Columbia, MD) ultraviolet–vis recording spectrophotometer with an extinction coefficient of 16,530 cm −1 M −1 at 280 nm. All protein purification steps were monitored by 4–12% Tris-Glycine SDS–PAGE (Lonza, Basel, Switzerland) to ensure they were virtually homogeneous. All chemicals and solvents were analytical and HPLC grade, respectively. Differential scanning fluorimetry (DSF) Purified p53 protein (0.22 mM in 50 mM HEPES at pH 7.5, 150 mM NaCl, 0.1 mM dithiothreitol) was diluted to 4 μM final concentration in 20 mM HEPES at pH 7.5. Compounds were dissolved in DMSO to various concentrations and added to diluted protein for overnight incubation at 4 °C. An equivalent volume of DMSO was used as a control and also incubated overnight at 4 °C. PRIMA-1 in DMSO was preheated at 90 °C for 20 min and cooled to room temperature before use [26] . Annexin A2, S100A4 and S100A10 were used as control proteins to rule out nonspecific interactions between compounds and p53. Sypro Orange stain (Bio-Rad, Hercules, CA) at 5,000 × stock concentration was diluted in 20 mM HEPES at pH 7.5 and added to each well for a final 5 × concentration. Each protein and compound condition was tested as replicates of 6 with 20 μl per well of a 96-well plate. DSF was performed on wild-type p53 and mutant G245S using the CFX96 Touch RT–PCR system (Bio-Rad) by increasing the temperature of the plate 0.5 °C per min from 25 to 52.5 °C. DSF performed on mutant R175H was identical except that the starting temperature was 10 °C. Fluorescence measurements were taken once every minute during all experiments. T m values for each well, mean T m values, and 95% confidence intervals were calculated with the program Prism 5 (GraphPad Software, La Jolla, CA) by fitting the raw fluorescence data to a Boltzmann sigmoidal curve. Accession codes: The coordinates of the human p53 core domain structures with the open binding pocket conformations have been deposited in the PMDB under accession codes PM0078199 for wt p53, PM0078200 for R175H, PM0078201 for G245S, and PM0078202 for R273H. How to cite this article: Wassman, C.D. et al. Computational identification of a transiently open L1/S3 pocket for reactivation of mutant p53. Nat. Commun. 4:1407 doi: 10.1038/ncomms2361 (2013).